Submicron structures provide preferential spots for carbon and nitrogen sequestration in soils The sequestration of carbon and nitrogen by clay-sized particles in soils is well established, and clay content or mineral surface area has been used to estimate the sequestration potential of soils. Here, via incubation of a sieved (<2 mm) topsoil with labelled litter, we find that only some of the clay-sized surfaces bind organic matter (OM). Surprisingly, <19% of the visible mineral areas show an OM attachment. OM is preferentially associated with organo-mineral clusters with rough surfaces. By combining nano-scale secondary ion mass spectrometry and isotopic tracing, we distinguish between new labelled and pre-existing OM and show that new OM is preferentially attached to already present organo-mineral clusters. These results, which provide evidence that only a limited proportion of the clay-sized surfaces contribute to OM sequestration, revolutionize our view of carbon sequestration in soils and the widely used carbon saturation estimates. Soils and marine sediments represent one of the largest reservoirs of organic carbon (OC) on Earth [1] , [2] , [3] and have a crucial role in global trace gas cycles and the associated climate change. In addition to occluding OM in aggregated mineral particles [4] , [5] , soils and sediments sequester OC and organic nitrogen (ON) through the formation of strong associations between OM and mineral surfaces in organo-mineral associations [6] , [7] . The association between OM and clay-sized particles accounts for a large proportion of sequestered OC in soils [8] . Clay-sized particles provide a multitude of reactive mineral surfaces for OC and ON binding [8] . The OC sequestration capacity of a soil is estimated from correlations between OC concentration and the soil’s clay content or specific surface area (SSA) [9] . Physical fractionation by density and/or particle size [8] is widely used to isolate organo-mineral associations. Understanding the dynamics of OM binding within the mineral matrix is essential for understanding the processes controlling the quantity, quality and turnover of OM attached to mineral particles [8] . Early research on marine sediments proposed a monolayer coverage of OM on clay mineral surfaces, as indicated by an indirect method (surface area calculations derived from N 2 adsorption measurements) [10] . However, techniques for direct investigation at the appropriate spatial scale are required for a better understanding of the relationship between organic structures and mineral grains [8] , [11] and of the spatiotemporal dynamics of the relationship. Direct analyses by transmission electron microscopy challenged the monolayer coverage concept and suggested that OM exists in patches associated with mineral surfaces [12] , [13] , which was confirmed by several other studies [14] , [15] , [16] , [17] , [18] . Synchrotron-based analyses showed highly complex forms of OM and reactive mineral materials interacting at the submicron scale [19] , [20] . To understand and quantify the OM sequestration potential of soils and sediments, the dynamics of OC and ON accumulation at the micro-scale must be studied. The key technique for tracking the biogeochemical cycles of C and N is stable isotope labelling ( 13 C, 15 N). Nano-scale secondary ion mass spectrometry (NanoSIMS) enables the direct visualization of 13 C and 15 N down to a lateral resolution of 150 nm [21] , [22] and can be used to identify organo-mineral associations by the simultaneous detection of ion species derived from the organic (C, N) and inorganic (Al, Si and Fe) components of the associations [18] , [23] , [24] , [25] . Here, our objective is to identify and quantitatively assess the OM-reactive surfaces in organo-mineral associations that control the C and N sequestration potential of soils. An incubation experiment over 42 days with an arable topsoil of a Luvisol (sieved to <2 mm) with 15 N- and 13 C-labelled litter is performed to quantify and follow the formation of organo-mineral associations. The soil chosen represents a type of soil common for central Europe, USA and south-east Australia with a mineral composition (illite, chlorite, mixed-layer clay minerals and pedogenic iron oxides) typical for the temperate zone. Microbial biomass- 13 C, salt-extractable OC- 13 C and isotopic C and N composition are determined for total bulk soil and selected soil fractions (which are obtained by combined density and particle size fractionation). The spatial distributions of mineral particles, OM and isotopic enrichment are investigated by NanoSIMS. Using this approach, we quantify the associations of OC and ON with mineral surfaces and identify hot spots of OM binding and label accumulation. Our data show that only some of the clay-sized mineral surfaces, namely those with rough surfaces, react with OM and thus contribute to OC and ON sequestration. Furthermore, these rough surfaces are the nuclei for additional OM accumulation and therefore, control the C and N sequestration potential of the soil. Thus, our results indicate that using the amount of clay as a proxy to predict the sequestration potential of soils and sediments is not sufficient. Accordingly, we propose that the contribution of these reactive surfaces must be quantified. Formation of new organo-mineral associations During our short-term incubation (42 days), the 13 C enrichment in the bulk soils decreased significantly ( U -test; P ≥0.05), from 0.89 to 0.67 atom-% ( Supplementary Table S1 , Supplementary Fig. S1a ). At 2 h after the start of the incubation, samples with added labelled litter already contained twice as much microbial biomass as the control samples ( Supplementary Table S2 ), pointing to enhanced microbial activity. The progression of litter decomposition was reflected by a linear decrease in C/N ratio ( Supplementary Fig. S1b ), a decrease in salt-extractable OC (SEOC) ( Supplementary Fig. S2 ), and a strong correlation between microbial biomass and 13 C concentration in the bulk soil ( r =0.88; P <0.001). Fresh, litter-derived 15 N and 13 C were found in all the fine mineral fractions shortly after start of the incubation experiment ( Fig. 1 ). Over the course of the incubation period, 13 C concentrations in the fine mineral fractions decreased ( Supplementary Table S3 ). In particular, the clay-sized fractions were more enriched in 15 N and 13 C compared with the other fine mineral fractions ( Fig. 1 ). 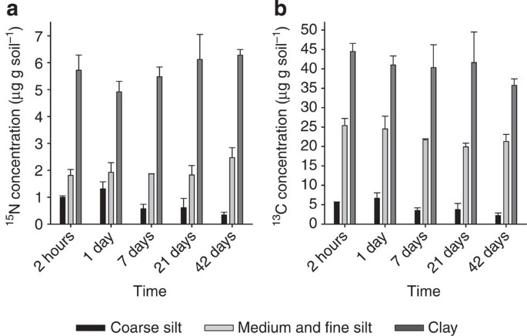Figure 1: Quantitative15N and13C enrichment in the fine mineral fractions. (a)15N and (b)13C concentrations (means, error bars indicate SDs,n=3) were calculated from the15N and13C excess values (obtained by IRMS) in the fine mineral fractions over the incubation time. Figure 1: Quantitative 15 N and 13 C enrichment in the fine mineral fractions. ( a ) 15 N and ( b ) 13 C concentrations (means, error bars indicate SDs, n =3) were calculated from the 15 N and 13 C excess values (obtained by IRMS) in the fine mineral fractions over the incubation time. Full size image Hot spots of OM sequestration in submicron soil structures To get insight into the spatial distribution and temporal development of freshly associated OM on clay-sized particles, we used scanning electron microscopy (SEM) and NanoSIMS to analyse the clay-sized fraction at four time points during the incubation period. SEM analysis revealed that some mineral particles appeared as individual particles with mostly plain surfaces, whereas others were aggregated in clusters of several small particles. This clustering causes rough surfaces. The surface roughness of mineral particles due to etch pits, micropores and cracks is generally defined as the ratio of the actual surface area to the surface of a hypothetical smooth surface enveloping the actual surface [26] . By SEM, we designated the mineral particles as either individual particles with plain surfaces or as clustered particles with rough surfaces ( Fig. 2a ). Hereafter, we refer to both the surface roughness due to etch pits, micropores and cracks and the observed roughness due to the clustering of mineral particles as ‘rough surface’. 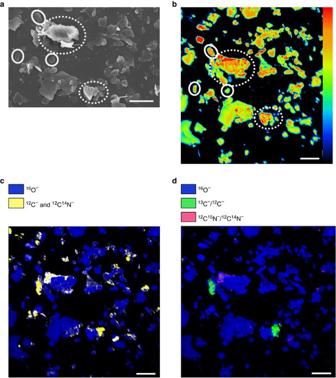Figure 2: New insights via two-dimensional NanoSIMS imaging. (a) SEM image and (b)16O−secondary ion image (linear 0–5191) of a representative clay-sized fraction (time point: 21 days) reveal individual (continuous circle) and clustered (dotted circles) particles. (c) The total OM, as revealed by12C−and12C14N−secondary ion images, on the mineral surfaces represents the organo-mineral associations. (d) The new, litter-derived OM is indicated by areas of the mineral surface where the13C−/12C−and12C15N−/12C14N−ratios were enriched compared with the ratios for the unlabelled clay-sized fraction. All scale bars represent 5 μm. Figure 2: New insights via two-dimensional NanoSIMS imaging. ( a ) SEM image and ( b ) 16 O − secondary ion image (linear 0–5191) of a representative clay-sized fraction (time point: 21 days) reveal individual (continuous circle) and clustered (dotted circles) particles. ( c ) The total OM, as revealed by 12 C − and 12 C 14 N − secondary ion images, on the mineral surfaces represents the organo-mineral associations. ( d ) The new, litter-derived OM is indicated by areas of the mineral surface where the 13 C − / 12 C − and 12 C 15 N − / 12 C 14 N − ratios were enriched compared with the ratios for the unlabelled clay-sized fraction. All scale bars represent 5 μm. Full size image We applied for the first time an approach of quantifying the areas visible by NanoSIMS. For each clay-sized fraction and time step, 10–12 spots (40 × 40 μm 2 each) were measured. These spots represented a total particle area of 5,815–9,474 μm 2 ( Table 1 ), which is more than 10 times the particle area analysed in previous studies of submicron-sized soil particles [24] . Of the total particle area, 13–26% was assigned to individual particles, and 74–87% was assigned to clustered particles ( Table 1 ). Consequently, in the analysed clay-sized fractions, most of the mineral particles were present in small clusters comprising rough surfaces. The mineral particles are displayed in the NanoSIMS images as 16 O − secondary ion images ( Fig. 2a ). All the OM, which was revealed by the 12 C − and 12 C 14 N − secondary ion images, was associated with mineral particles, and the OM was heterogeneously distributed in small patches on the particles ( Fig. 2b ). By linking the images for OM and for the mineral particles, we found that only 1–2% of the individual particles were covered by OM, whereas 15–21% of the mineral clusters contained OM ( Table 1 ). Determination of the SSA by N 2 adsorption showed that, in particular, mineral particles with a large SSA were covered by OM. We calculated that about 77% of the total SSA was covered by OM ( Supplementary Table S4 ). Table 1 Quantification of exposed two-dimensional areas visible by NanoSIMS. Full size table Organo-mineral clusters as nuclei for new OM sequestration We used 13 C − / 12 C − and 12 C 15 N − / 12 C 14 N − ratios obtained by means of NanoSIMS to evaluate the spatial distribution of newly incorporated OM in the clay-sized fractions. To follow the changes in the new, litter-derived OM, we quantified as new OM areas where the 13 C − / 12 C − and 12 C 15 N − / 12 C 14 N − ratios were enriched compared to the values for the unlabelled clay-sized fraction. Figure 2c shows spots enriched in 13 C and 15 N, demonstrating distinct micro-scale hot spots of new labelled OM. The 13 C − / 12 C − and 12 C 15 N − / 12 C 14 N − ratios measured for numerous spots by NanoSIMS showed a much higher variability in comparison to the isotope ratio mass spectrometry (IRMS) data, indicating a high spatial heterogeneity of the sample ( Fig. 3 ). 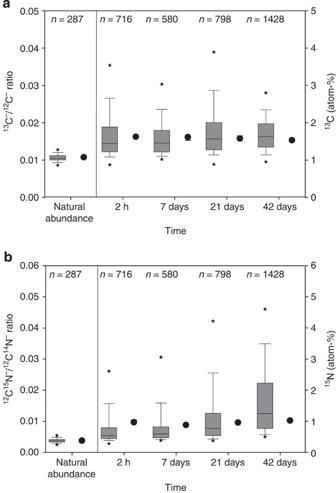Figure 3: Heterogeneity of newly formed organo-mineral associations. (a) Box plots of13C−/12C−ratios obtained by NanoSIMS reflecting the number of evaluated regions of interest (ROIs) (medians, error bars indicate data range within 5th and 95th percentiles) and13C values (dots) obtained by IRMS (medians, error bars indicate SEs, n=3). (b)12C15N−/12C14N−ratios obtained by NanoSIMS reflecting the number of evaluated ROIs (medians, error bars indicate data range within 5th and 95th percentiles) and15N values (dots) obtained by IRMS (medians, error bars indicate SEs,n=3). Outliers are marked with asterisks. The ratios for an unlabelled clay-sized fraction were used to prove enrichment and are called natural abundance. Figure 3: Heterogeneity of newly formed organo-mineral associations. ( a ) Box plots of 13 C − / 12 C − ratios obtained by NanoSIMS reflecting the number of evaluated regions of interest (ROIs) (medians, error bars indicate data range within 5th and 95th percentiles) and 13 C values (dots) obtained by IRMS (medians, error bars indicate SEs , n =3). ( b ) 12 C 15 N − / 12 C 14 N − ratios obtained by NanoSIMS reflecting the number of evaluated ROIs (medians, error bars indicate data range within 5th and 95th percentiles) and 15 N values (dots) obtained by IRMS (medians, error bars indicate SEs, n =3). Outliers are marked with asterisks. The ratios for an unlabelled clay-sized fraction were used to prove enrichment and are called natural abundance. Full size image The data obtained by NanoSIMS were generally on the same order of magnitude as the bulk IRMS values ( Fig. 3 ). Most of the isotopically enriched spots (94–96%) showed enrichment in both 13 C and 15 N isotopes, whereas the rest of the enriched spots showed enrichments in either 13 C or 15 N ( Table 1 ). We assume that the spots enriched in 13 C and 15 N ( Fig. 2c ) represent new OM formed during the incubation experiment, whereas spots that show no enrichment represent pre-existing OM. By overlaying the spots showing total OM ( Fig. 2b ) with the enriched spots ( Fig. 2c ), we were able to differentiate spots with old and new labelled OM. The areas enriched in 13 C and 15 N as a proportion of the total OM area increased from 33–55% during incubation ( Table 1 ), whereas the total OM area changed only marginally over time. Our IRMS data demonstrate the fast formation of new organo-mineral associations in addition to the organo-mineral associations already present from the original soil material. This is because of the rapid decomposition of the added litter. The presence of fresh litter-derived 15 N and 13 C in the fine mineral fractions point to an immediate incorporation [27] . This incorporation is not solely caused by sorption processes, but also due to microbial activity, which is indicated by the small C/N ratio in the clay fraction suggesting that the chemical composition is dominated by microbial residues and metabolites [8] ( Supplementary Table S3 ). Our quantitative NanoSIMS results reveal for the first time that almost all the OM existing in the clay-sized fraction was bound in mineral clusters. The rough surfaces of clustered particles might provide preferential binding sites for OM [13] . The results of the SSA determination ( Supplementary Table S4 ) indicate that especially small mineral particles with a high surface roughness got covered by OM, which confirms our findings by NanoSIMS. The OC loading of 1.1±0.1 mg m −2 determined for the clay-sized fractions ( Supplementary Table S4 ) fell into the range proposed for the monolayer coverage [9] , [28] , [29] . However, because the clustered particles contained most of the OM, these organo-mineral clusters exhibited a much higher capacity for OC storage than expected for a monolayer. We demonstrated for the first time that small mineral particles with rough surfaces in organo-mineral clusters provide the essential reactive interfaces for OM sequestration. Our results clearly indicate that mineral particles with a smooth surface are not suited for substantial OM sequestration, presumably because they do not have etch pits, micropores or cracks. Preferential OM sequestration on mineral clusters with rough surfaces also might be due to better hydration and nutrient conditions at rough surfaces, conditions that offer an advantageous microhabitat for microorganisms [30] . Using our approach of visualizing and quantifying the exposed surfaces, we discovered that most of the mineral surfaces did not show any OM coverage at all. Clay content is often used as a proxy for the estimation of a soil’s OC sequestration potential [9] , [31] . These findings may explain why clay content is sometimes poorly related to OC concentration [32] . The heterogeneity of organic patches on mineral surfaces observed by NanoSIMS is generally not detected by bulk IRMS soil analyses [25] . Synchrotron-based near-edge X-ray spectromicroscopy of mineral assemblages illustrated that OM is present in extremely heterogeneous forms, such as plant or microbial biopolymers, at distinct locations [20] . The increased variability in the detected 12 C 15 N − / 12 C 14 N − ratios might have been caused by fractionation of protein-rich microbial metabolites during the interaction of OM with mineral surfaces [33] . The organic spots that were enriched in both isotopes represent OM bound to mineral surfaces derived either directly from the litter or from the microbial products originating from litter decomposition. The area enriched solely in 15 N increased from 2 to 5% during the incubation period ( Table 1 ). From the accumulation of such OM enriched only in 15 N, we infer that this represents material that was more intensively processed by microbes. Thus, NanoSIMS provides detailed insight into the spatial variability of OM accumulation during such an incubation experiment. At the end of the incubation, the isotopic labels were extensively incorporated over about half of the organo-mineral cluster areas. This high proportion of areas covered with new labelled OM was unexpected on the basis of the enrichments measured for the clay fraction by IRMS, representing only about 44 μg 15 N and 310 μg 13 C per gram of clay-sized fraction, but is explained by the observation that <19% of the total mineral area is covered by OM. Our findings indicate a preferential attachment of new OM to organo-mineral clusters with rough surfaces containing pre-existing OM. This is demonstrated by an increase of area enriched in 13 C and 15 N, while the total area covered with OM remains constant ( Table 1 ). Our data are in agreement with a conceptual model of preferential sorption of OM on surfaces already containing sorbed OM [34] , [35] . Although we could assign a large proportion of the total area in the clay-sized fractions to individual smooth mineral particles or clusters (80%), they did not contribute to binding of new OM. This result implies that only a limited proportion of the total clay-sized mineral particles were involved in OM sequestration. This finding was unexpected because the clay-sized mineral particles in this soil (illite, mixed-layer clay minerals and pedogenic iron oxides, such as goethite) are all considered to be reactive on all surfaces owing to their permanent and variable charges ( Supplementary Fig. S3 ). These findings have major implications for our understanding of fundamental soil properties that are controlled by the surface reactivity of the fine soil fraction, such as cation exchange capacity, pollutant binding capacity and physical properties. Our data also point to the necessity for careful identification and quantification of the reactive mineral complexes that are responsible for OM sequestration and that control the OM saturation capacity of soils and sediments. Such data could be incorporated into current models for estimating the carbon sequestration capacity of soils and can be expected to considerably improve the predictive power of such models. Soil and litter characterisation For the incubation experiments, we used soil from the uppermost 5 cm of the Ap horizon, a lamellic Luvisol (raptic, arenic and bathygleyic, according to IUSS Working Group WRB soil classification system [36] ). The soil had an organic C content of 13.5±0.9 mg g −1 , a N content of 1.4±0.0 mg g −1 , a C/N-ratio of 9.6±0.4 and a pH value of 5.5±0.1. The natural abundance for 13 C and 15 N in the soil were 1.075 and 0.369 atom-%. The clay, silt and sand contents were 18.5%, 18.4% and 63.0% ( Supplementary Table S5 ). The oxalate-extractable iron content was 21.2±0.0 mg g −1 , and the dithionite-extractable iron content was 62.8±2.3 mg g −1 . The mineral composition of the clay fraction was dominated by chlorite, illite, quartz and mixed-layer minerals, as indicated by X-ray diffraction ( Supplementary Fig. S3 ). The litter we used was derived from a 1:1 mixture of maize ( Zea mays ) and potato ( Solanum tuberosum ) dried leaf material. The unlabelled litter had an organic C content of 405.2±1.9 mg g −1 , a N content of 23.7±0.1 mg g −1 and a C/N-ratio of 17.1±0.1. The 15 N and 13 C contents of the unlabelled litter were 0.396 and 1.084 atom-%. A mixture of unlabelled litter and soil was used to determine the natural abundances of the bulk soil and the soil fractions. The labelled litter had an organic C content of 404.2±1.8 mg g −1 , a N content of 23.3±0.0 mg g −1 and a C/N-ratio of 17.3± 0.1. The 15 N and 13 C concentrations were 6.1 and 4.9 atom-%, respectively. Experimental design We thoroughly mixed 50 g of sieved soil (<2 mm) with 0.5 g of litter (<200 μm). Three treatments were incubated: (1) labelled litter and soil (three independent replicates), (2) unlabelled litter and soil (three independent replicates) and (3) an additional treatment per time point without litter, as a control. After litter addition, the soils were incubated for 42 days under defined conditions at 14 °C and at 60% maximal water holding capacity. To maintain the water content, we moistened the soil columns at 2 day intervals. Samples were taken at five time points during incubation: after 2 h and after 1, 7, 21 and 42 days. Bulk analyses For the determination of SEOC, a 5 g aliquot of fresh soil was shaken with 20 ml of 0.01 M CaCl 2 for 45 min, and then the suspension was filtered (Whatman, grade 595 ½, Bruchsal, Germany). SEOC in the filtrate was determined on a total carbon analyser (DIMATOC 2000, Dimatec Analysen GmbH, Essen, Germany) by catalytic high-temperature oxidation. Microbial biomass (C mic ) was determined according to the fumigation–extraction method [37] . A 5 g aliquot of fresh soil was extracted with 0.01 M CaCl 2 , as described for SEOC measurements. C mic was calculated as the difference between C total in fumigated (fum) and non-fumigated (n-fum) samples using a k EC value of 0.45 (ref. 38 ). Atom-% 13 C in the extracts was measured via online liquid chromatography coupled with stable IRMS (MAT 253, Thermo Fisher Scientific, Dreieich, Germany) [39] . The atom-% 13 C in microbial biomass (atom-% 13 C mic ) was computed as where 13 C fum and 13 C n-fum are atom-% 13 C values of the fumigated and non-fumigated extracts, respectively, and C fum and C n-fum are the respective carbon concentrations [40] . For further analyses, the bulk soil was dried at 40 °C. Aliquots were ground and homogenized with a vibrating ball mill with zircon-grinding tools (Pulverisette 23, Fritsch, Germany). OC, 13 C, N and 15 N were determined in duplicate by means of an isotope ratio mass spectrometer (Delta V Advantage, Thermo Fisher Scientific, Dreieich, Germany) coupled to an elemental analyser (Euro EA, Eurovector, Milan, Italy). Appropriate standards were included for normalization correction, instrument linearity and precision [41] . Values of 15 N and 13 C atom-% excess were calculated by subtracting 13 C and 15 N enrichment of the respective soil with unlabelled litter from the corresponding enrichments obtained for the treatments with labelled litter. All calculated contents were determined from the atom-% excess values. Physical soil fractionation To remove all free labelled litter and to extract the organo-mineral associations, we conducted a combined density and particle size fractionation. Dry soil material (30 g, <2 mm) was saturated with 300 ml of sodium polytungstate solution (density 1.8 g cm −3 ) and allowed to settle overnight. The floating free particulate organic matter fraction (fPOM) was removed by means of a water jet pump. For disruption of the soil aggregates, the remaining slurry was ultrasonically dispersed (Sonopuls HD 2200, Bandelin, Germany; VS 70 T Sonotrode Ø 13 mm with a liquid coverage of 1.5 cm) with an energy input of 450 J ml −1 . Subsequently, the dispersed sample was centrifuged (15 min at 3019 × g ) to separate the occluded particulate OM from the mineral residue. To remove the sodium polytungstate from the fPOM and occluded particulate OM, the fractions were washed with deionized water on a pressure filtration unit (Durapore Membrane Filters, pore size 0.22 μm, Millipore, Switzerland). The remaining organo-mineral fraction was centrifuged several times with deionized water until the electrical conductivity was <50 μS cm −3 . The mineral residues were wet-sieved at 63 μm and 20 μm mesh sizes to separate the sand and coarse silt fractions, respectively. The soil material fraction of <20 μm was separated into medium and fine silt (20–2 μm) and clay (<2 μm) via sedimentation. All fractions were dried (40 °C) and weighed to obtain the mass proportion of each fraction relative to the bulk soil. We analysed fPOM and the smaller mineral fractions (coarse, medium and fine silt, and clay) for OC, 13 C, N and 15 N as described above for the bulk soil. Values of 13 C atom-% and 15 N atom-% excess were calculated by subtracting the values for the respective fractions of unlabelled soil (fractions of soil with unlabelled litter) from the enrichments obtained from the labelled fractions for each time point. Specific surface area The SSA of the clay-sized fraction was determined using a standard method for measuring surface area in soils based on the physisorption of N 2 gas on a sample at 77 K using the Brunauer–Emmett–Teller equation [42] . Nitrogen adsorption was measured at 11 points in the partial pressure range of 0.05–0.3 with an Autosorb-1 analyser (Quantachrome, Syosset, NY, USA). Before measurement, the samples were outgassed for 14–20 h in vacuum under helium flow at 40 °C. The SSA was measured for the clay-sized fraction before and after OM removal to assess the coverage of SSA by OM [15] . OM was removed by oxidation with a 10% H 2 O 2 solution at room temperature. NanoSIMS analysis Clay-sized fractions at the time points of 2 h and 7, 21 and 42 days, as well as a clay-sized fraction with unlabelled litter as natural abundance, were analysed by means of NanoSIMS (Cameca NanoSIMS 50l, France). A 1 mg sample of dried clay-sized fraction was dispersed in 20 ml of deionised water, and 100 μl of the dispersion was dropped on a silica wafer, which was dried overnight in a desiccator. The homogeneous distribution of the particles was checked with a reflected-light microscope (Axio Imager Z2m, Zeiss, Germany). Reflected-light microscopic images of the whole sample were taken for documentation and later orientation on the sample using the CCD camera of the NanoSIMS. SEM images (Jeol JSM-5900LV, Eching, Germany) were taken to support interpretation of the NanoSIMS results. Prior to SEM measurements, the samples were coated with gold (~5 nm; SCD 005 sputter coater, Bal-tec GmbH, Germany) to avoid charging. For NanoSIMS analysis, the Cs + primary ion probe was used with a primary ion impact energy of 16 keV. Prior to analysis, contaminants and an additional gold coating layer (~30 nm) were sputtered away by a high primary beam current (pre-sputtering). During the pre-sputtering, the reactive Cs + ions were implanted into the sample to enhance the secondary ion yields. The primary beam (~1.2 pA) focused at a lateral resolution of 100–200 nm was scanned over the sample (40 × 40 μm), and 12 C − , 13 C − , 12 C 14 N − , 12 C 15 N − , 16 O − and 27 Al 16 O − secondary ions were collected on electron multipliers with an electronic dead time fixed at 44 ns. The estimated depth resolution with 16 keV Cs + ions as primary ion beam is about 15 nm. The measurements were performed at high mass resolving power to circumvent the occurrence of mass interferences (for example, 12 C 1 H − versus 13 C − , 12 C 14 N − versus 12 C 2 1 H 2 − and 12 C 15 N − versus 13 C 14 N − ). We compensated for the charging due to the non-conductive mineral particles by using the electron flood gun of the NanoSIMS instrument. All measurements were done in imaging mode. The ion images were acquired using a dwell time of 1–3 ms/pixel, 512 × 512 pixels and one cycle. For every sample, 10–12 spots were analysed to obtain a reliable data basis for the calculation of the fate of 13 C and 15 N. NanoSIMS images were evaluated using the Open MIMS Image plugin for the ImageJ software. All images were corrected for electron multiplier dead time (44 ns). ROIs were chosen according to the distribution of the 12 C − and 12 C 14 N − secondary ions as an OM indicator. The threshold option of the ImageJ software was used to automatically generate the ROIs for these images. For this, the triangle algorithm was used [43] . The ROIs of the 12 C − and 12 C 14 N − images were combined afterward to obtain the ROIs for the OM distribution. Areas and sums of secondary ion counts for each ROI were extracted from all images. All ROIs with an area greater than 10 pixels were used for further calculations. Mineral particles were selected as ROIs on the basis of 16 O − and 27 Al 16 O − images. For structural analyses, the visible mineral surface areas were divided into clustered particles and individual particles on the basis of the corresponding SEM images. Data presentation and statistical analysis Mean values and standard deviations were calculated using Microsoft Excel (2007). IRMS data were statistically analysed with IBM SPSS Statistics (ver. 19.0, IBM, Armonk, NY, USA). For this analysis, the means of three independent replicates were tested using a non-parametric test ( U -test) with a significance level of 95%. Figures were prepared and regressions were performed with SigmaPlot software (ver. 11.0, Systat Software, Erkrath, Germany). How to cite this article: Vogel, C. et al. Submicron structures provide preferential spots for carbon and nitrogen sequestration in soils. Nat. Commun. 5:2947 doi: 10.1038/ncomms3947 (2014).